Allostery through the computational microscope: cAMP activation of a canonical signalling domain Ligand-induced protein allostery plays a central role in modulating cellular signalling pathways. Here using the conserved cyclic nucleotide-binding domain of protein kinase A’s (PKA) regulatory subunit as a prototype signalling unit, we combine long-timescale, all-atom molecular dynamics simulations with Markov state models to elucidate the conformational ensembles of PKA’s cyclic nucleotide-binding domain A for the cAMP-free (apo) and cAMP-bound states. We find that both systems exhibit shallow free-energy landscapes that link functional states through multiple transition pathways. This observation suggests conformational selection as the general mechanism of allostery in this canonical signalling domain. Further, we expose the propagation of the allosteric signal through key structural motifs in the cyclic nucleotide-binding domain and explore the role of kinetics in its function. Our approach integrates disparate lines of experimental data into one cohesive framework to understand structure, dynamics and function in complex biological systems. Since the introduction of the allosteric effect in L -threonine deaminase [1] , [2] , researchers have sought to understand the mechanisms of allostery. The classical phenomenological models proposed by Monod–Wyman–Changeux [3] and (Pauling)–Koshland–Nemethy–Filmer [4] , [5] have been extended over time to emphasize population shifts or modulations in the conformational ensemble of the proteins [6] , [7] . Fundamentally, it is the character of the underlying free-energy landscape that determines the mechanism of allostery [6] , [7] , [8] , [9] , [10] , [11] . While experimental and computational approaches provide insight into allosteric mechanisms [12] , [13] , a robust atomic-level description of the free-energy landscape remains a challenge due to a variety of methodological limitations. Without an atomic-level description of the conformational ensemble and its corresponding free-energy landscape, the details of allostery can remain hidden within ensemble averages or constrained perspectives of protein conformation and dynamics. The objective of our work is to apply cutting-edge computational approaches to explore the conformational ensemble of a protein with and without a bound ligand, thereby gaining insight into how the ensemble gives rise to protein function. This work focuses on the mechanism of ligand-driven allostery in the cyclic nucleotide-binding domain of protein kinase A’s (PKA) regulatory subunit. Despite extensive research conducted on this system [14] , questions still remain. The intercellular activation of PKA by cAMP is a prototypical example of ligand–protein allostery, which occurs through the cooperative binding of cAMP to tandem cyclic nucleotide-binding domains, designated A and B, in each of PKA’s regulatory subunits [14] . Crystallographic data show that the regulatory subunit, isoform Iα, undergoes significant conformational changes on binding cAMP. It transitions from an extended holoenzyme conformation that inhibits PKA’s catalytic subunits to a compact cAMP-bound conformation that releases and activates PKA’s catalytic subunits [15] , [16] . Within the cyclic nucleotide-binding domain, the inactive holoenzyme and the active cAMP-bound conformations of the regulatory subunit are characterized by the conformational changes in three structural motifs—the N3A motif, the phosphate-binding cassette (PBC) and the B/C helix [17] , [18] , leaving the core β-barrel subdomain largely unchanged ( Fig. 1 ). These structural motifs represent the fundamental signal transduction component and form the binding interface between the cyclic nucleotide-binding domain and PKA’s catalytic subunit. 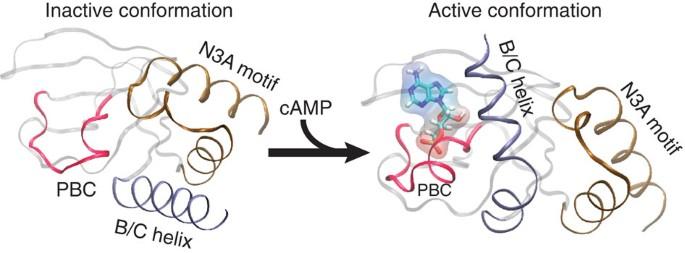Figure 1: Experimentally determined conformational changes in the cyclic nucleotide-binding domain. (RIα a.a. 119 to 244) in cAMP bound active, right and holoenzyme inactive, left, with key signalling structural subdomains highlighted: PBC, red; B/C helix, ice blue; and N3A motif, ochre. Figure 1: Experimentally determined conformational changes in the cyclic nucleotide-binding domain. (RIα a.a. 119 to 244) in cAMP bound active, right and holoenzyme inactive, left, with key signalling structural subdomains highlighted: PBC, red; B/C helix, ice blue; and N3A motif, ochre. Full size image The existing crystallographic data provide only two conformational states for the cyclic nucleotide-binding domains, the holoenzyme (a.k.a. H or inactive) [16] , [19] and the cAMP-bound conformation (a.k.a. B or active) [15] . Nuclear magnetic resonance (NMR) dynamics data of the minimal functional component of PKA’s regulatory subunit, the A cyclic nucleotide-binding domain (a.a. 119–244), indicate the presence of two dominant conformational states [20] , [21] , [22] and suggests conformational selection as the mechanism of allostery [23] . On cAMP binding, changes in NMR chemical shift data implicate the PBC as a major dynamic element, while few changes are observed in the N3A motif or the B/C helix. However, such experiments are limited in their ability to elucidate details of the full structural ensemble. Instead, they provide averaged metrics that correlate to dynamic motions. Achieving an atomistic description of the underlying conformational ensemble and resolving the corresponding free-energy landscape will clarify the mechanisms by which cAMP modulates the function of the cyclic nucleotide-binding domain. Because the PKA holoenzyme contains four cyclic nucleotide-binding domains, cAMP-induced activation is a complicated process. A recent study by Boras et al . [24] provided a general blueprint of the events during activation at the subcellular level, but the molecular mechanism of activation remains to be elucidated. To build a foundation on which to address these questions, we simulated fully solvated atomistic models of the conformational ensembles of the A cyclic nucleotide-binding domain (hereafter referred to as the cyclic nucleotide-binding domain or CBD), with and without cAMP bound. Extensive molecular dynamics (MD) simulations were integrated using Markov state model theory to explore PKA’s conformational space and long-timescale dynamics. Markov state models depict the interaction dynamics of discrete interconnected states as a transition probability matrix, at a fixed lag time, assuming that the transitions between the states are independent of previous transitions (that is, Markovian) [25] , [26] , [27] , [28] . By assigning individual frames extracted from MD trajectories to discrete conformational states, sampling from many separate trajectories can be integrated into one coherent framework that captures the kinetics and thermodynamics of the conformational ensemble at atomic resolution. Similar approaches have been used to study protein folding [29] , biased transition pathways between functional states [30] , [31] , identification of cryptic allosteric sites [32] and ligand regulation of G-protein-coupled receptors [33] . Our work is unique in that it directly assesses the atomic conformational landscape using initial unbiased long-timescale MD simulations augmented with adaptive sampling of one protein in two functional states, as opposed to only combining many short-timescale simulations or sampling along a predetermined reaction coordinate. We find that the conformational ensembles of cAMP-free (CBD–Apo) and cAMP-bound (CBD–cAMP) functional states exist within a shallow free-energy landscape that allows access to both experimentally determined functional conformations, indicating conformational selection as the principal mechanism of allostery with the isolated cyclic nucleotide-binding domain. We find that the addition of cAMP modifies the principal motions of the cyclic nucleotide-binding domain, which correspond to transitions between active and inactive states. Furthermore, our approach exposes the propagation of the allosteric signal through the cyclic nucleotide-binding domain’s signalling motifs. Our results complement existing structural [15] , [16] and dynamical [20] , [21] , [22] , [23] , [34] experimental data, and extend our understanding of the mechanism of ligand-induced allostery within the cyclic nucleotide-binding domain. Further, they provide a general framework for understanding the function of the ancient and ubiquitous cyclic nucleotide-binding domain [35] , [36] and allosteric mechanisms more generally. Modelling the conformational landscape To explore and map the conformational landscapes of the cyclic nucleotide-binding domain, we integrated multiple MD simulations with Markov state models. Explicit solvent MD simulations of the cyclic nucleotide-binding domain were performed with and without cAMP-bound systems (CBD–cAMP and CBD–Apo, respectively). The MD simulations of both systems sampled a totalled 74 μs ( Supplementary Table 1 ). The simulations were composed of four long-timescale, ∼ 13-μs simulations on the Anton supercomputer [37] (at the Pittsburgh Supercomputing Center) and multiple parallel short-timescale, 0.5–1 μs simulations using GPU-accelerated AMBER12 (refs 38 , 39 , 40 ). For both systems, sampling simulations were initiated from experimentally determined atomic coordinates of the cyclic nucleotide-binding domain [15] , [16] in both the inactive and active conformations. Initial sampling was followed by multiple rounds of directed sampling (10–15 ns simulations using GPU-accelerated AMBER12 (refs 38 , 39 , 40 )) to refine the Markov state models [41] . Directed sampling simulations were initiated from intermediate conformations selected near poorly sampled transitions within the Markov state model. For both the CBD–cAMP and CBD–Apo systems, no single simulation sampled a complete transition between the experimentally determined inactive and active structures. However, simulations started from either experimental conformation overlapped in conformational space, based on alpha carbon root mean squared distance (r.m.s.d. ), indicating that the MD trajectories could be integrated meaningfully into a single Markov state model ( Supplementary Fig. 1 ). To build the Markov state models, we needed to define the conformational space, and then divide the space into discrete conformational states. As in protein-folding models [29] , the cyclic nucleotide-binding domain conformations are defined by the atomic coordinates of each residue’s alpha carbon. We divided the sampled conformational space into discrete conformational states through r.m.s.d. clustering using MSMBuilder2 (ref. 42 ). We prealigned the structures to a common reference frame to calculate r.m.s.d. to capture important translational motions lost using the standard minimum r.m.s.d. approach, which aligns each pair of compared structures to each other before determining r.m.s.d.. Inspection of the individual MD trajectories indicated that the β-barrel of the cyclic nucleotide-binding domain was stable relative to the motions of the N3A motif, the PBC and the B/C helix ( Supplementary Fig. 2 ). Therefore, we used the β-barrel as our common reference frame. All conformations sampled from the MD simulations of both the CBD–Apo and CBD–cAMP systems were clustered together to create a comprehensive framework of conformational states. Once the conformation states were identified, Markov state models were built for each system. This means that the models were built using the same division of conformational space, but each model included only states sampled in its respective simulations. (A comparison between this approach and clustering conformations from CBD–Apo and CBD–cAMP separately is discussed below.) The Markov state models were built by specifying the maximum distance or cutoff for the clustering algorithm, which determined how the conformational space was divided, and a lag time for the model. Model parameters were selected because they were Markovian, as indicated by implied timescale plots, and could maximize the number of conformational states. In addition, consistency between the Markov state models and the MD simulations were determined by the Chapman–Kolmogorov test [26] (that is, were the models’ generated trajectories similar to the results from the original MD simulations? ; Supplementary Figs 3–10 ). An evaluation of several r.m.s.d. cutoffs and lag times indicated that the best Markov state model utilized a clustering cutoff of 3.0 Å and a lag time of 9.6 ns ( Supplementary Figs 3 and 4 ). Graphs of the Markov state models for CBD–Apo and CBD–cAMP are visualized as a network ( Fig. 2 ). Each node corresponds to a cluster of similar conformations or a single conformational state. The diameters of the nodes are proportional to the log of equilibrium population of the conformational state. Thus, smaller nodes indicate conformations that are more rarely sampled. The location of each node is determined by the r.m.s.d. of the structure of the cluster’s generator, approximately the centroid of the cluster, to the inactive and active crystallographic structures. We note that the location of each node gives a general indication of the conformation of each state relative to the experimental structures, but node locations are a projection from a higher-dimensional space. (Separation of the experimentally determined active node, indicated in Fig. 2 , from the bulk of the other nodes is an artifact of the clustering algorithm in MSMBuilder2 (ref. 42 ), which selects the first MD frame (that is, the equilibrated starting active conformation) as a generator for the first cluster. Notice that the separation of the active conformation node from its neighbours is ∼ 3 Å or the r.m.s.d. cutoff of the clustering algorithm.) 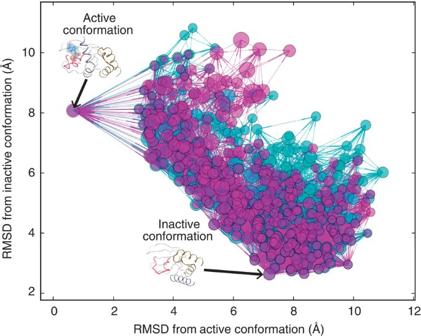Figure 2: Overlay of Markov State Models State Graphs for the cyclic nucleotide-binding domain with (CBD–cAMP, magenta) and without (CBD–Apo, cyan) cAMP bound. The position of each conformational state node is the r.m.s.d. of the generator of each cluster relative to the reference conformations. The diameter of each conformational state node (cyan, magenta) is proportional to the relative the log of the equilibrium population. (that is, the lager the node the more probable the state at equilibrium.) Cyan and magenta nodes are transparent; therefore, dark purple nodes represent nodes that have occupancy in both CBD–Apo and CBD–cAMP Markov state models (that is, dark purple nodes overlap). Figure 2: Overlay of Markov State Models State Graphs for the cyclic nucleotide-binding domain with (CBD–cAMP, magenta) and without (CBD–Apo, cyan) cAMP bound. The position of each conformational state node is the r.m.s.d. of the generator of each cluster relative to the reference conformations. The diameter of each conformational state node (cyan, magenta) is proportional to the relative the log of the equilibrium population. (that is, the lager the node the more probable the state at equilibrium.) Cyan and magenta nodes are transparent; therefore, dark purple nodes represent nodes that have occupancy in both CBD–Apo and CBD–cAMP Markov state models (that is, dark purple nodes overlap). Full size image Ligand-meditated changes in the conformational ensemble A comparison of the models of the conformational state ensembles for the CBD–Apo and CBD–cAMP systems allowed us to assess how the binding of cAMP modifies the overall free-energy landscape. We compared the distribution of conformational states between the two systems, the overall character of the free-energy landscape and the kinetics of traversing the free-energy landscape between functional conformations states. For this comparison, and throughout this work, we assumed that the crystallographic structures represent the functional conformations (active or inactive states) of the cyclic nucleotide-binding domain. The nodes containing the functional conformations are indicated in Fig. 2 . When comparing the conformational landscapes of CBD–Apo and CBD–cAMP, we noticed two striking features—the large number of shared states ( Fig. 2 ) and the character of the unique states. The models indicate that the systems share ∼ 70% of the total number of sampled conformational states ( Supplementary Table 2 ). Notably, the shared conformational states of CBD–Apo and CBD–cAMP comprise 66 and 38%, respectively, of the total population for each ensemble. Many of the unique CBD–Apo conformational states contain structures in which the cAMP-binding site is formed poorly and, thus, sterically prevented from occurring when cAMP is bound ( Supplementary Fig. 11 ). Many of the most populated unique CBD–cAMP conformational states exhibit structures in which the C terminus is interacting with cAMP ( Supplementary Fig. 12 ). These states include the dynamical capping of cAMP’s adenosine ring by Y244, part of the C-helix, which substitutes the native capping residue W260 from the ‘B’ CBD in the full regulatory subunit [15] , [43] . These capping interactions with Y244 have been observed experimentally in the truncated RIα (a.a. 1–259) [43] but not previously observed in simulations. In addition, fluorescent experiments studying the dynamics of R239 (located on the C-helix) indicate that the C-helix has a higher propensity to interact with the core cyclic nucleotide-binding domain in the presence of cAMP [34] . The unique CBD–cAMP conformational states are not sterically excluded from the CBD–Apo conformation ensemble, and interactions between the C terminus and the cAMP-binding sites were observed in the CBD–Apo ensemble. Therefore, the absence of unique states in the CBD–cAMP ensemble is likely due to the absence of stabilizing interactions between cAMP and the C terminus. Importantly, both models sampled the active and inactive states; yet, neither state is the most populated conformational state in either system. Using the most probable conformational state as the reference state, at physiological conditions, the depth of free-energy landscape is 6.6 kcal mol −1 for CBD–Apo and 7.6 kcal mol −1 for CBD–cAMP. The free energies for the individual conformational states follow a Gaussian distribution with a mean depth of the free-energy landscape at 3.1±1.4 kcal mol −1 for CBD–Apo and 4.2±1.6 kcal mol −1 for CBD–cAMP. The transition free energy out of a conformational state to any of its neighbouring conformational states (that is, only states that it is connected to) ranges from 5.8 to 8.6 kcals mol −1 for both systems. (5.8 kcal mol −1 corresponds to a transition made at approximately the lag time of the Markov state model and, thus, is the lowest bound transition free energy calculated from the Markov state model.) The absolute difference in free energy between the active and inactive states is 0.1 kcal mol −1 for CBD–Apo and 0.9 kcal mol −1 for CBD–cAMP. Overall, the free-energy landscapes of both systems provide access to both functional states at physiological conditions, with cAMP binding deepening the free-energy landscape by ∼ 1 kcal mol −1 . Transition pathway theory [44] , [45] identified the 10 highest flux paths between the functional conformational states for each ensemble ( Supplementary Fig. 13 ). 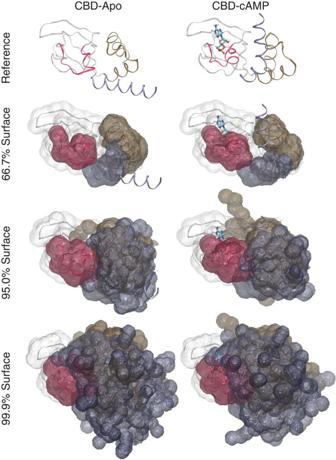Figure 3: Equilibrium probability density surfaces for CBD–Apo and CBD–cAMP at 66, 95 and 99.9% cutoffs. The surfaces correspond to the probability density surface for each residues alpha carbon. Densities contributed from key structural subdomains are coloured: PBC, red; B/C helix, ice blue; and N3A motif, ochre. SeeFig. 1for the description of CBD representations. The proportion of the highest flux path relative to the total flux for each functional state ensemble was striking: For CBD–Apo, the highest flux path was only 9% of the total flux, and for CBD–cAMP, it was only 4% of the total flux ( Supplementary Table 3 ). The lack of a dominant path and the variety of paths identified in the analysis indicate that there are multiple pathways between functional conformational states. Inspection of the pathways indicated no common order of conformational changes or shared features at the bottlenecks of the pathways. Therefore, to understand the transition between active and inactive conformation states across the free-energy landscape, we needed to look at the transition pathways collectively. We measured the kinetics of the transition between active and inactive states using mean first passage times (that is, the fastest average time it takes for the system to move across the free-energy landscape from active-to-inactive state, or vice versa; Table 1 ). Interestingly, the mean first passage times for the transition from inactive to active state are similar with or without cAMP bound: ∼ 30 μs. However, the addition of cAMP slows the transition from active-to-inactive state by a factor of five, from 16 to 84 μs. Table 1 Mean first passage time between active and inactive conformations. Full size table These results indicate that CBD–Apo favours the inactive state, which inhibits PKA’s catalytic subunit, whereas CBD–cAMP favours the state that activates PKA’s catalytic subunit. Thus, the dynamics of the cyclic nucleotide-binding domain derived from the Markov state models are consistent with the function of the regulatory subunit in PKA. Taken together, our results indicate conformational selection as the governing mechanism of allostery in the cyclic nucleotide-binding domain. The weakest evidence for this mechanism is the number of shared states between both models because it is largely a function of the clustering algorithm. However, when the conformations for each system are clustered separately, the results are the same. In fact, the joint clustering approach better captures the principal motions of the CBD at a 3.0-Å clustering cutoff, as determined by implied timescale plots ( Supplementary Fig. 14 ). The stronger evidence supporting conformational selection is the change in the free-energy landscape and the corresponding transition kinetics. Weinkam et al . [8] classified allosteric mechanisms based on the difference between the change in free energy of two functional states and the binding free energy of the ligand. Although the current Markov state models do not allow determination of the free energy of cAMP binding, and there has been no direct experimental measurements of cAMP binding in our construct, we can estimate the binding free energy of cAMP through previous work on the isolated A cyclic nucleotide-binding domain [46] . The free energy of binding of cAMP to the isolated A cyclic nucleotide-binding domain is ∼ −3 kcal mol −1 (ref. 46 ). This value is greater than the difference in free energy between the active and inactive states, ∼ −1 kcal mol −1 , supporting conformational selection as the general mechanism of allostery. In addition, the on-rate for cAMP to the A cyclic nucleotide-binding domain of R, ∼ 4.8 × 10 4 s −1 (ref. 46 ), is faster than the transition times between active and inactive states in the CBD–cAMP system. And the fact that the transition rates between inactive and active conformations are independent of ligand binding indicate conformational selection as described by Zhou [9] . Experimental results [23] , [47] support conformational selection as the mechanism of ligand-induced allostery, thus complementing the interpretations of our Markov state model presented here. One limitation of our model is the potential bias towards conformational selection because the simulations were initiated at both experimentally determined active and inactive states, which were included in and connected through the Markov state models. However, nothing sterically hinders cAMP from binding either functional conformational state in the absence of the catalytic subunit, and no restraints were required to keep cAMP bound during the simulations. Thus, all four systems used to initiate the simulations are potential members of the conformational ensemble. Starting the simulations in each experimental conformation does not predispose them to becoming members of highly populated or networked states or bias the transition kinetics between active and inactive states. Details of the allosteric mechanism While our results indicate conformational selection as the general mechanism of allostery for the CBD, this finding is not wholly novel due to previous experimental work [23] , [47] . However, our work provides a foundation to delve further into the mechanisms of allostery at an atomic scale in ways inaccessible to current experimental methods: we can explore structural characteristics of the equilibrium conformational space, and the principal motions of the CBD and its functional macrostates. To understand the structural characteristics of the conformational landscapes, we built stationary probability density volumes of the positions of the alpha carbons. In other words, we sought to determine the probability of finding the mass of the alpha carbons in a given volume of space at equilibrium. The volumes were determined by dividing the space in 0.1 Å voxels and calculating the probability of finding an alpha carbon within 3 Å (the r.m.s.d. cutoff for the Markov state model) of the voxel for each conformational state. By summing over all states, we obtained a map of the stationary probability density, which provides a visual representation of the conformational ensembles. Fig. 3 shows the probability of density surfaces at 66, 95 and 99.9%. The volume enclosed by each surface has a probability greater than the cutoff of being occupied by an alpha carbon. This figure shows the wide range of motion sampled by the α-helical structural subdomain at equilibrium; this range of motion is similar for the CBD–Apo and CBD–cAMP systems. Similar to the graphical representation of the Markov state model, the stationary probability density volumes indicate the similarity of the conformations sampled by CBD–Apo and CBD–cAMP. Figure 3: Equilibrium probability density surfaces for CBD–Apo and CBD–cAMP at 66, 95 and 99.9% cutoffs. The surfaces correspond to the probability density surface for each residues alpha carbon. Densities contributed from key structural subdomains are coloured: PBC, red; B/C helix, ice blue; and N3A motif, ochre. See Fig. 1 for the description of CBD representations. Full size image However, the differences between the stationary probability density volumes give us new structural insight into the mechanisms of allostery within the CBD. The first notable difference is the unique density formed by the B/C helix proximal to cAMP in the CBD–cAMP ensemble ( Fig. 4a ). This density corresponds to the interactions between the C terminus and the adenosine ring of cAMP discussed above. A second difference is the higher probability that the N3A motif extends over the B/C helix in the CBD–Apo ensemble ( Fig. 4b ). This density corresponds with the experimentally determined binding interface between PKA’s catalytic and regulatory subunits [16] . Interestingly, the CBD–Apo system only increased density by about 10% in forming the interface. This small variation shows how seemingly small changes in a conformation ensemble give rise to inhibitory function of the CBD–Apo system by increasing the probability of formation of the binding interface between PKA’s catalytic and regulatory subunits. 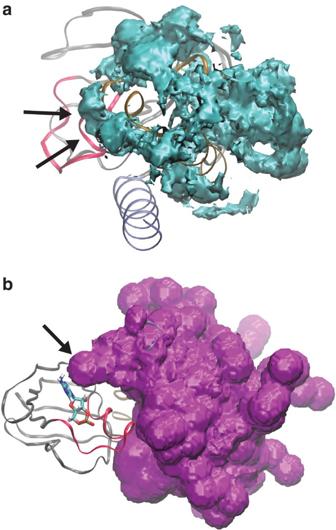Figure 4: Selected difference surfaces between equilibrium probability densities of CBD–Apo and CBD–cAMP. (a) The difference surface for 10% or more density for the N3A Motif of CBD–Apo over CDB–cAMP. Arrows indicate interface between PKA’s catalytic and regulatory subunits (b) The different surface for 1% or more density for the B/C Helix of CBD–Apo over CDB–cAMP. Figure 4: Selected difference surfaces between equilibrium probability densities of CBD–Apo and CBD–cAMP. ( a ) The difference surface for 10% or more density for the N3A Motif of CBD–Apo over CDB–cAMP. Arrows indicate interface between PKA’s catalytic and regulatory subunits ( b ) The different surface for 1% or more density for the B/C Helix of CBD–Apo over CDB–cAMP. Full size image To determine the principal motions of the CBD, we built kinetic coarse-grained models from the Markov state models of each system to identify metastable states or the principal motions of CBD arising from the conformational ensemble. These models were generated by complementarily employing principal component and Markov clustering analysis [25] , [28] , [32] , [42] , [48] , [49] . The CBD–Apo implied timescale plots ( Supplementary Fig. 3 ) suggest at least one dominant slow motion followed by numerous secondary faster motions. The dominant slow motion of the CBD–Apo ensemble is between conformations similar to the active and conformations similar to the inactive conformational states ( Fig. 5 ). Of note, the second most dominant motion is integration of the unfolded N-helix (the N3A motif) into the core β-barrel ( Supplementary Fig. 15 ). These conformations are only observed in the CBD–Apo ensemble as they deform the cAMP-binding site, sterically excluding cAMP. Integration of the unfolded N-helix requires partial unfolding of the core β-barrel, which was observed in previous NMR work [21] . We recognize that these conformations may be an artifact of the truncated CBD and, therefore, may not be part of the mechanisms of allostery for the regulatory subunit in vivo . Still, the consistency between the results of the simulations and the NMR work indicates that the models are able to replicate structural events seen experimentally. 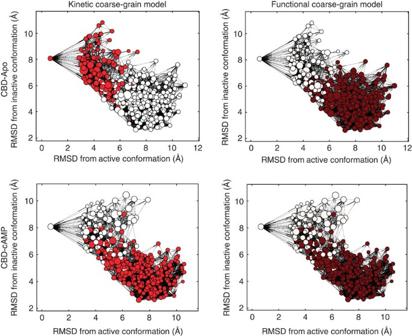Figure 5: Comparison of conformational state assignment for kinetic and functional coarse-grain models. Conformational state metastable states for the first/slowed motions in the kinetic coarse-grain Markov state model graph are coloured below according to macrostate membership (red, white). Functional coarse-grain models are coloured either white or maroon, depending on whether the state ‘would go’ to the active or inactive conformations, respectively. Figure 5: Comparison of conformational state assignment for kinetic and functional coarse-grain models. Conformational state metastable states for the first/slowed motions in the kinetic coarse-grain Markov state model graph are coloured below according to macrostate membership (red, white). Functional coarse-grain models are coloured either white or maroon, depending on whether the state ‘would go’ to the active or inactive conformations, respectively. Full size image Like the CBD–Apo system, the implied timescale plot for the CBD–cAMP system indicates one dominant slow motion followed by a number of faster motions ( Supplementary Fig. 4 ). Although the dominant motion is structurally similar to that of CBD–Apo (that is, it is also the transition between active and inactive conformations ( Fig. 5 )), it is slower than that of CBD–Apo (compare Supplementary Figs 3 and 4 ). Interestingly, the second slowest motion within the CBD–cAMP system corresponds to those states where the C terminus is interacting with cAMP. To strengthen the relationship between motions of the CBD and its function, we generated a functional coarse-grained model of the conformational ensembles. The model identifies which conformational stats have a higher probability of transitioning to either the active of inactive state, thus indicating the role of each conformational state in the function of the system. Using committer analysis from transition pathway theory [44] , [45] , the ensembles were divided into two functional macrostates. Each macrostate was composed of conformational states with a >50% probability of transitioning to the active or inactive state. In other words, the functional coarse-grain model can be conceptualized as the ‘continental divide’ of the free-energy landscape, indicating to which functional state (active or inactive) an individual conformational state is connected to most strongly. The functional coarse-grain model of CBD–Apo ( Fig. 4 ) contains similar populations for the active and inactive macrostates, with a preference for the inactive macrostate. CBD–cAMP ( Fig. 4 ), however, prefers the active macrostate ( Table 2 ). These results agree with NMR studies that show similar inactive and active conformational populations at very-low-cAMP concentration and domination of the active macrostate at high-cAMP concentrations [21] . In addition, the relationship of the half-life of either functional macrostate is similar to the mean first passage time between functional conformational states in that transitions from inactive to active states have similar kinetics in both systems, whereas the presence of cAMP slows the transition from active to inactive state ( Table 2 ). Table 2 Population and half-life for CBD–Apo and CBD–cAMP coarse-grain functional states. Full size table The functional coarse-grain model and the kinetic coarse-grain model closely correlate with each other as determined by conformational state membership in the functional or kinetic macrostates. Correlation between the two coarse-grained models is expected as they both depend on the transition kinetics of the Markov state models; however, which motion corresponded to the change in functional states is not clear a priori. This correlation indicates that the functional macrostates determined by transition pathway theory correspond to the slowest motion of the cyclic nucleotide-binding domain ( Fig. 4 ). It also supports the assumption that the crystallographic conformations represent the active and inactive states of the cyclic nucleotide-binding domain and that its slowest motion is the transition between active and inactive states. The coarse-grained models combined with observations of the change in stationary probability densities for the two systems support a general explanation that the modification of the transition kinetics by cAMP gives rise to function. In CBD–Apo, transitions between states occur with a tendency towards the inactive conformation, which increases the likelihood of generating the interface that allows for the regulatory subunit to bind the catalytic subunit leading to inactivation of PKA. With cAMP bound, the transition between inactive and active states is slower, which is likely the result of interactions formed between the C terminus and cAMP. The preference for the active-like conformations in the CBD–cAMP system decreases the probability of forming the binding interface and allowing activation of PKA. Motions of the signalling motifs To gather more detail on the allosteric mechanism, we examined the propagation of an allosteric signal through the helical signalling motifs of the cyclic nucleotide-binding domain by building new Markov state models for the three principal signalling motifs using the same MD trajectories (apo and cAMP-bound). While the motions of the signalling motifs are captured in the Markov state models of the full CBD, as discussed above, individual models elucidate the conformational ensembles of focused structural elements and provide an unobstructed view of their modulation by cAMP. The Markov state models for the individual motifs were developed and analysed using the same methods for the full system ( Supplementary Figs 5–10 ). They indicate conformational selection as the general mechanism of allostery, due to well-connected active and inactive conformational states ( Fig. 6 ) with multiple pathways across the free-energy landscape for each of the three key motifs ( Supplementary Table 3 ). 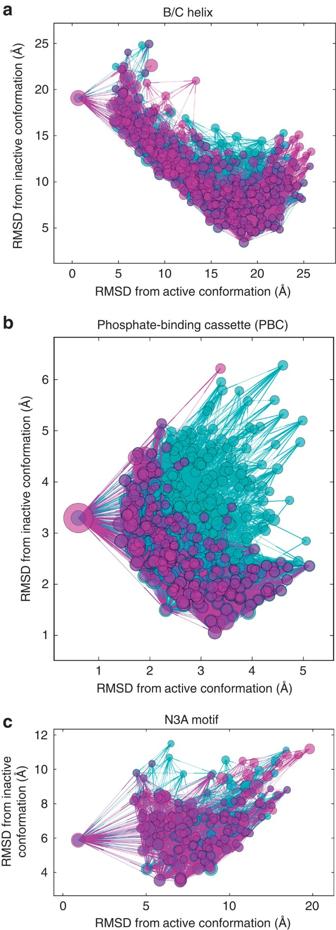Figure 6: Overlay of Markov State Model Conformational State Graphs for the SubDomains of cyclic nucleotide-binding Domain with (CBD–cAMP, magenta) and without (CBD–Apo, cyan) cAMP Bound. Markov state models conformational state graphs use the same conventions defined inFig. 2. Figure 6: Overlay of Markov State Model Conformational State Graphs for the SubDomains of cyclic nucleotide-binding Domain with (CBD–cAMP, magenta) and without (CBD–Apo, cyan) cAMP Bound. Markov state models conformational state graphs use the same conventions defined in Fig. 2 . Full size image When we compared the conformational state distribution between the apo and cAMP-bound systems, we observed that the N3A motif and the B/C helix share a majority of their conformational states ( Fig. 6 and Supplementary Table 2 ), similar to the full cyclic nucleotide-binding domain. The B/C helix generally explores the conformational space between the experimentally determined active and inactive structures ( Fig. 6a ). However, the N3A motif explores conformations dissimilar to either experimental conformation ( Fig. 6c ). These models are consistent with the observed motions of these domains ( Supplementary Fig. 2 ), particularly with the unfolding of the N-helix ( Supplementary Fig. 11 ). These results support and help explain why there is no observed change in chemical shifts in NMR experiments [21] for the N3A motif or the B/C helix despite the changes in the crystallographic structures ( Fig. 1 ). Simply put, in solution the conformational space explored by the N3A motif and the B/C helix is largely independent of cAMP, though cAMP does modulate the relative populations of the conformational states and their kinetics. In contrast, the PBC showed significant changes in chemical shifts on binding cAMP [21] . While these changes appear to be driven by interaction with cAMP, the Markov state model of the PBC illuminates another aspect of these changes: that, on binding of cAMP, the PBC loses about half of its conformational states, representing a significant loss in conformational entropy ( Fig. 6b , Supplementary Table 2 ). In addition, the kinetic and functional coarse-grain models of the PBC show significant changes between apo and cAMP systems ( Supplementary Fig. 17 and Supplementary Table 5 ) unlike the other signalling motifs ( Supplementary Figs 16 and 18 and Supplementary Tables 4,6 ). Without cAMP, the PBC has a shallow free-energy landscape with quick transition between metastable macrostates ( Table 1 , Supplementary Fig. 17 , and Supplementary Table 5 ). With cAMP bound, there is one dominant (slow) transition between two metastable macrostates ( Table 1 , Supplementary Fig. 17 and Supplementary Table 5 ; also compare implied timescale plots in Supplementary Figs 7 and 8 ). Unlike the other models ( Fig. 5 and Supplementary Figs 16 and 18 ), the conformational states that comprise these metastable macrostates do not correspond to the division of microstates seen in the functional coarse-grain model ( Supplementary Fig. 17 ). Instead the functional coarse-grain model indicates a strong propensity of the PBC to assume a cAMP-binding conformation or active conformation even in the absence of cAMP ( Supplementary Fig. 17 and Supplementary Table 5 ). Overall, the model shows that, without cAMP bound, the PBC explores a variety of conformations, but the binding site has a tendency to assume the active cAMP-bound conformation. cAMP binding selects the active conformation while allowing transition between active and inactive state but significantly slows the transition between these states ( Table 1 , Supplementary Table 5 ). The spatial arrangement of the helical signalling motifs suggests that the propagation of the allosteric signal would be from the PBC to the B/C helix to the N3A motif ( Fig. 1 ). Even the natures of the conformation ensembles, described by the Markov state models, suggest propagation of the allosteric signal from a switch like the PBC out to the conformationally diverse N3A motif. However, the kinetics of the signalling motifs suggest another mechanism. The mean first passage times between active and inactive states suggest that the movement of the B/C helix is the rate-limiting step for the functional transition because it has the slowest transitions between active and inactive states ( Table 1 ). Like the full CBD, the B/C helix has similar transition times between active and inactive states whether or not cAMP is bound. However, cAMP significantly decreases the rate of the active-to-inactive transition ( Table 1 ). This rate reduction is due to the stabilization of the active conformation by cAMP through interactions between the C helix and cAMP ( Fig. 4 ), as observed and discussed above. In PKA and other proteins, the experimental free energy of binding of cAMP to the cyclic nucleotide-binding domain is dominated by enthalpic contributions [50] , [51] , [52] , suggesting that the contacts between cAMP and the PBC and B/H helix are drivers for this phenomenon. Our model indicates that the binding of cAMP near the PBC dampens the dynamics of that signalling motif, greatly increasing its propensity to adopt an active-like conformation, and that the motions of the B/C helix are the rate-limiting step in this transition. Overall, we find that the prototype cyclic nucleotide-binding domain is a highly dynamic system and that cAMP modulates its function by modifying the dynamics of the signalling motifs. By comparing CBD–Apo and CBD–cAMP ensembles, we see that the free-energy landscape allows access to both active and inactive states through an ensemble of transition pathways (that is, there is no one dominant pathway between states). Collectively, our analysis supports conformational selection as the general mechanism of allostery in this system. The addition of cAMP modulates the transition rates between the functional states but only between active-to-inactive states and not vice versa. This modulation of rates occurs by slowing motion in the CBD–cAMP ensemble, which is caused by interactions with cAMP. Finally, our work indicates that the change in dynamics of the B/C helix is the rate-limiting step in adopting a fully active conformation. Furthermore, the motion of the B/C helix is essential for signal propagation to the N3A motif and formation of the interface with the catalytic subunit. This mechanism could be tested experimentally though NMR by observing shifts in the relative populations of active and inactive ensembles caused by mutations in the C terminus, specifically, mutations of residue 244, which should modify interactions with cAMP. While the general mechanism of allostery for the cyclic nucleotide-binding domain is conformational selection, some elements of the mechanism appear to behave more like induced fit. Particularly notable in this regard are the interactions between the C-helix and cAMP, which generate multiple conformational states that are not sampled in the apo state, as compared with the motions of the individual signalling motifs that appear more similar to entropic mechanisms of allostery. Furthermore, in the context of activation of the full kinase, these mechanisms may change, as interaction with the catalytic subunit and the remaining portions of the regulatory subunit will almost certainly modulate the conformational ensemble of the cyclic nucleotide-binding domain. This work suggests that a clearer picture of the free-energy landscape, achieved through an integrated experimental and computational approach, is required to fully understand allosteric behaviour. Although a number of our conclusions were already observed experimentally, the power of our computational Markov-state-model-based approach is that it unifies multiple lines of existing experimental data into a single, cohesive framework and, thereby, achieves a more complete understanding of allostery. This approach builds on an emerging paradigm for understanding protein function and dynamics based on computational exploration and visualization of protein conformational ensembles and their underlying functional free-energy landscapes in atomic detail. System preparation Parameterization of cAMP . We parameterized cAMP for the MD simulations as a small organic molecule using the generalized amber force field [53] to allow for consistent treatment of ligands in future studies. The coordinates for cAMP were taken from the 1RGS [15] crystal structure. Partial atomic charges for cAMP were determined by single-point energy calculations using Schrodinger’s QM module Jaguar (Suite 2012: Jaguar, version 7.9, Schrödinger, LLC, New York, NY, 2012) using the Hartree–Fock level of theory and 6-311g** bases. Generalized amber force field atom types were assigned using antechamber [54] , and the parameters files were prepared with AMBER’s xleap. MD System preparation . Using Schrodinger’s Maestro’s (Suite 2012: Maestro, version 9.3, Schrödinger, LLC, New York, NY, 2012) PDB prep and the Desmond System Preparer, we prepared four systems for MD simulations, CBD–Apo and CBD–cAMP in both the active and inactive conformations. The heavy-atom atomic coordinates for the active and inactive conformations of CBD–Apo were taken for crystal structures 1RGS [15] and 2QCS [16] resides 119 to 244, respectively. We added cAMP to the inactive conformation by aligning the cAMP-binding site of 1RGS and 2QCS and ‘cutting and pasting’ the coordinates. For the CBD–Apo active conformation, the coordinates for cAMP were deleted from 1RGS. Within PBD prep, each system was capped to remove terminal charges, the systems were protonated at pH 7.0 with the pK a titratable residues determined with the Maestro-integrated PROPKA, and, due to the low resolution of 1RGS, all crystallographic waters were removed. Using the Desmond System Preparer, we solvated each system in a cubic water box using TIP3 waters [55] , counter ions, and 120 mM NaCl. No restraints were placed on cAMP. MD simulations System parameterization . System coordinates from Maestro were converted into an xleap-readable format using in-house Python scripts. Each system was parameterized in xleap using the Amber99SB [56] force field and periodic boundary conditions were implemented. GPU-enabled MD simulations . All systems were minimized and equilibrated using the GPU version of Amber12 (refs 38 , 39 , 40 ). We minimized the system in four stages: (1) 500 steps of hydrogen-only minimization, (2) 500 steps of solvent minimization, (3) 500 steps with only the backbone constrained and (4) 5,000 steps of full minimization. We equilibrated the system using harmonic equilibration at 310 K over four sequential 500-ps runs, decreasing the restraint potential on the backbone each step. GPU-enabled AMBER12 production runs were carried out as an NTP ensemble at 310 K and 1 bar with a 2-fs time-step and partial mesh Ewald electrostatic approximation. MD input files are provided as part of the data sharing. Anton MD simulations . MD simulations on Anton [37] were performed on the same parameterized, minimized and equilibrated systems as GPU-enabled AMBER12 simulations. The Anton simulation was run in the NTP ensemble, using Anton’s Berendsen thermostat-barostat, at 310 K and 1 bar with a 2-fs time-step and partial mesh Ewald electrostatic approximation. Initial and adaptive sampling . We sampled the conformational ensemble from the equilibrated conformation of each system, starting each run with a different set of initial velocities. Supplementary Table 1 contains the total sampling time for each system used in this analysis. In conjunction with model building, we performed multiple adaptive sampling runs. These runs were initiated from preliminary Markov state model conformational states with <3 members. These conformational states corresponded to clustered regions of the conformational ensemble poorly sampled by the MD simulations and, therefore, the transitions to and from those states were poorly sampled. For each under-sampled conformational state, one conformation was selected. From that conformation, three new 10–15 ns MD simulations were run, each with a new initial velocity using GPU-enabled AMBER12. The short MD simulations were sufficient to explore the local conformational landscape and return to a local energy minimum. Building Markov state models Trajectory preparation . MD trajectories were processed using CPPTRAJ [57] and VMD [58] . All frames were aligned using Cα of residues 153 to 199 and 211 to 223, the stable β-barrel, to crystallographic active conformation. The alignment provided a common reference frame to compare all conformations while maximizing the difference between conformations. The frame rate for the trajectories was unified to 120 ps due to different conformational sampling rates between the GPU-enabled AMBER12 (0.5 ps) and Anton (120 ps) MD simulations. The trajectories were converted into NAMD’s [59] ‘.dcd’ trajectory format for analysis with MSMBuilder2. Building the Markov State Model . We used MSMBuilder2 (refs 32 , 42 ), release 2.51, to preform cluster analysis, Markov state model building and Markov state model selection. To have a common set of microstates for both the CBD–Apo and CBD–cAMP systems, all trajectories were clustered together using the hybrid k-centres k-medoids clustering algorithm using the custom distance metric option to calculate r.m.s.d. without first performing an alignment on the atomic coordinates (an option not available in MSMBuilder2). MSMBuilder2 allows for refinement of clustering through refinement of frame membership within a cluster as well as global refinement of cluster generators. For our systems, we found that any refinement only made the space discretization worse, as determined by implied timescale plots. Therefore, we didn’t use any refinement options for our clustering. Markov state models were then built on the CBD–Apo and CBD–cAMP trajectories separately using cluster generators to assign state membership to each frame of the trajectories. When the best conformational landscape partition and lag time were determined (see discussion below), a final Markov state model was built using the maximal likelihood estimator option in MSMBuilder2. Model selection . For the Markov state model of the whole systems, we selected a clustering cutoff distance of 3.0 Å and a lag time of 80 steps or 9.6 ns. For consistency in comparing models, a lag time of 9.6 ns was used for all. Markov state model visualization . The Markov state models were visualized using in-house Python scripts leveraging the publically available NetworkX module [60] . Markov state model analysis Equilibrium population . The equilibrium population was determined from the first eigenvalue of the Markov state model’s transition probability matrix that corresponds to the equilibrium distribution of the conformational states. Transition pathway theory analysis . Transition pathway theory analysis was preformed using MSMBuilder2 transition pathway theory scripts [42] . Total flux was calculated as described in Prinz et al . [45] . Transition pathway theory-based clustering was preformed using in-house Python scripts leveraging MSMBuilder2 modules. The script assigned transition pathway theory macrostates to each microstate of the original Markov state model based on the probability of transitioning to either the inactive or the active conformation (cutoff 50%). The conformational state assignments for each frame of the trajectories were reassigned using in-house Python scripts and a new Markov state model based on the macrostate assignments was built with MSMBuilder2. Markov cluster analysis macrostate models . Markov cluster analysis clustered the states of the Markov state model based on their kinetic relationships within the Markov state model using a random walk algorithm to determine local sinks in the Markov state model [48] . We performed the Markov cluster analysis using in-house Python scripts that assigned new Markov cluster analysis state assignments to the original state assignments and built a Markov state model. In addition, we used MSMBuilders2’s PCCA+ (ref. 42 ) module to validate the division identified through Markov clustering. Mean first passage time . Absolute MFPT between the putative functional microstates was calculated as described in Singhal et al . [61] Half-life The half-life of coarse-grained microstates was calculated using a kinetic Monte Carlo scheme on the Markov state model’s transitions matrix as described in Shukla et al . [31] Trajectories were generated by randomly selecting a starting state within a macrostate, then moving between states based on the transition’s probability as determined by the Markov state model. The passage time of the trajectory was the number of steps in the trajectory multiplied by the lag time (9.6 ns). The half-life was calculated by taking the average of 10 median passage times from a collection of 1,000 trajectories. Calculating kinetics and free energies . Assuming that transitioning out of one conformational state into its neighbouring conformational states can be modelled as parallel reactions, we can treat the kinetics for the conformational changes between connected conformational states as first-order reactions. Therefore, we determined the rate constant using where k in the first-order rate constant, p 0 is the probability of starting in a given state (that is, the starting concentration or 1), p 1 is the probability of still being in that state at a given lag time (that is, the concentration after a give time) and τ is the lag time (9.6 ns). The free energy of transition was calculated using Eyring’s equation as follows: where R is the gas constant, h is Plank’s constant, k B is Boltzmann’s gas constant, κ is the transmission coefficient assumed to be 1, T is temperature (310 K) and k is the rate constant calculated above. The free energy of a single microstate was calculated using where is the probability of a given microstate, p r is the probability of the reference microstate (the most probable microstate in the ensemble), R is the gas constant (0.0012, kcal mol −1 K −1 ) and T is temperature (310 K) [62] . Markov state model signalling motifs The Markov state models of the signalling motifs were built and analysed using the same methods described above except we only used a subset of Cα. The residues used for the analysis of each subdomain were: 119 to 151 for the N3A motif, 199 to 211 for the PBC and 226 to 244 for the B/C helix. Markov state models were built with a clustering cutoff of 4.5 Å for the N3A motif, 1.5 Å for the PBC and 4.5 Å for the B/C helix. The lag time used was 9.6 ns. Data sharing MD trajectories, sample MD input scripts and the Markov state model analysis scripts are available for download at http://dx.doi.org/10.6075/J0Z60KZS . How to cite this article: Malmstrom, R. D. et al . Allostery through the computational microscope: cAMP activation of a canonical signalling domain. Nat. Commun. 6:7588 doi: 10.1038/ncomms8588 (2015).